The CREB/CRTC2 pathway modulates autoimmune disease by promoting Th17 differentiation Following their activation in response to inflammatory signals, innate immune cells secrete T-cell-polarizing cytokines that promote the differentiation of naive CD4 T cells into T helper (Th) cell subsets. Among these, Th17 cells play a prominent role in the development of a number of autoimmune diseases. Although regarded primarily as an immunosuppressant signal, cAMP has been found to mediate pro-inflammatory effects of macrophage-derived prostaglandin E2 (PGE 2 ) on Th17 cells. Here we show that PGE 2 enhances Th17 cell differentiation via the activation of the CREB co-activator CRTC2. Following its dephosphorylation, CRTC2 stimulates the expression of the cytokines IL-17A and IL-17F by binding to CREB over both promoters. CRTC2-mutant mice have decreased Th17 cell numbers, and they are protected from experimental autoimmune encephalitis, a model for multiple sclerosis. Our results suggest that small molecule inhibitors of CRTC2 may provide therapeutic benefit to individuals with autoimmune disease. T helper 17 (Th17) cells promote clearance of pathogens such as Mycobacterium tuberculosis and Candida albicans [1] ; they are also implicated in autoimmune diseases such as multiple sclerosis, rheumatoid arthritis, inflammatory bowel disease and asthma. Following their activation, innate immune cells secrete cytokines such as transforming growth factor (TGF)-β and interleukin (IL)-6, which promote the differentiation of naive CD4 T cells into Th17 cells [2] , [3] , [4] . In turn, Th17 cells secrete factors such as IL-17A and IL-17F to recruit neutrophils and macrophages for pathogen clearance [5] . Both IL-17A and IL-17F appear critical for Th17 function, as mice deficient in these two cytokines are resistant to a mouse model of multiple sclerosis called experimental autoimmune encephalomyelitis (EAE) [6] , [7] . The paracrine hormone prostaglandin E2 (PGE 2 ) exerts both immunosuppressive and pro-inflammatory effects on immune cells. PGE 2 suppresses the function of macrophages, neutrophils, Th1 cells and natural killers, for example; yet it promotes Th2, regulatory T cell and Th17 cell responses [8] . PGE 2 has been found to function through Gs-coupled EP2 and EP4 receptors, which upregulate IL-17A and IL-17F expression [9] . Although PGE 2 concentrations are elevated in cerebrospinal fluid from multiple sclerosis patients, the role of this paracrine hormone in this setting is unknown [10] . Animal studies on EAE support a dual role for PGE 2 in promoting the generation of Th17 cells during immunization and in modulating entry of Th17 cells into the central nervous system (CNS) [11] . cAMP is thought to function primarily as an immunosuppressant signal; it inhibits nearly every pathway downstream of the T-cell receptor to suppress T-cell activation, proliferation and cytokine production [12] . Despite these effects, T cells deficient in cAMP signalling due to targeted disruption of the Gα unit of the heterotrimeric G protein show a block in Th17 cell differentiation and inflammatory responsiveness [13] . In line with these pro-inflammatory effects, the cAMP-responsive factor CREB has been found to enhance the activation, proliferation and survival of T-cells [14] . Mice deficient in CREB1 and the CREB family member, ATF-1, have reduced thymic cellularity and delayed recovery following sublethal irradiation [15] . Moreover, mice expressing a dominant-negative CREB polypeptide exhibit defects in proliferation, IL-2 production and impaired T-cell function [16] , [17] . In addition to promoting CREB phosphorylation, cAMP also stimulates cellular gene expression via the PKA-dependent dephosphorylation of the CRTC family of CREB co-activators. Sequestered in the cytoplasm under basal conditions, CRTCs translocate to the nucleus following their dephosphorylation, where they bind to CREB on relevant promoters [18] . Of the three family members, CRTC2 is abundantly expressed in the liver, spleen and lymph nodes ( http://biogps.gnf.org/ ). While the CREB–CRTC2 pathway has been shown to function importantly in glucose metabolism and B-cell differentiation, its role in T-cell development and function has not been fully characterized [19] , [20] . Here we use mice with a knockout of the CRTC2 gene to evaluate its effects on T-cell differentiation. Our results highlight an unexpected role for the CREB pathway in adaptive immunity. Th17 differentiation is defective in CRTC2-mutant mice We evaluated thymic phenotypes of CRTC2-mutant ( Crtc2−/−) mice compared with control littermates. The relative proportions of CD4 or CD8 single-positive, double-positive and double-negative thymocytes were similar between Crtc2−/− and control littermates ( Supplementary Fig. 1a ). Splenic CD4 and CD8 T-cell numbers were also comparable ( Supplementary Fig. 1b ). Although naive CD4 T cells from both groups differentiated comparably into Th1, Th2 and regulatory T (Treg) cells in vitro ( Fig. 1a,b ), the differentiation of Crtc2−/− cells into Th17 cells was significantly impaired ( Fig. 1b ); IL-17A ( il17a ) and IL17F ( il17f ) cytokine expression was also reduced in CRTC2 mutant relative to control ( Fig. 1c ). Consistent with these changes, mRNA amounts for il17a and il17f were also downregulated in Crtc2−/− CD4 T cells ( Fig. 1d ). Crtc2−/− Th17 cells also had lower mRNA amounts for NR4A2, a well-established CREB/CRTC2 target that has been shown to regulate Th17 differentiation and autoimmune disease ( Fig. 1d ) [18] , [21] . 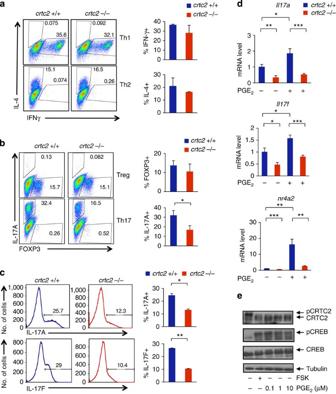Figure 1: Decreased Th17 differentiation in CRTC2-mutant mice. (a,b) Wild-type and CRTC2-mutant naive CD4 T-cells skewed towards Th1, Th2, Treg and Th17 cells. Cytokine levels determined using flow cytometry. Plots are gated on live CD4 T-cells. Number in each quadrant indicates cell frequency. Data are representative of three experiments. Bar graphs represent the mean of percentage (right)±s.e.m.,n=3, from three independent experiments with similar results. (c) Decrease in IL-17A and IL-17F secreting Th17 cells from CRTC2-mutant or wild-type littermates under Th17 differentiation conditions. IL-17A and IL-17F levels determined using flow cytometry. The electronic gate indicates the frequency of IL-17A (top) or IL-17F (bottom) CD4 T-cells. Data are representative of three experiments. Bar graphs represent the mean percentage (right)±s.e.m.,n=3, from three independent experiments with similar results. (d) mRNA amounts for IL-17A, IL-17F and NR4A2 in CRTC2-mutant T-cells under Th17 differentiation conditions. Treatment with PGE2indicated. Data represent the mean±s.e.m.2,n=3, from three independent experiments with similar results. (e) Immunoblot showing effect of PGE2and forskolin (FSK) on CRTC2 dephosphorylation and CREB phosphorylation in CD4 T-cells under Th17 differentiation conditions. Statistical analysis were performed with unpaired Student’st-test. Differences were considered statistically significant atP<0.05 (*P<0.05; **P<0.005 and ***P<0.0005). Figure 1: Decreased Th17 differentiation in CRTC2-mutant mice. ( a , b ) Wild-type and CRTC2-mutant naive CD4 T-cells skewed towards Th1, Th2, Treg and Th17 cells. Cytokine levels determined using flow cytometry. Plots are gated on live CD4 T-cells. Number in each quadrant indicates cell frequency. Data are representative of three experiments. Bar graphs represent the mean of percentage (right)±s.e.m., n =3, from three independent experiments with similar results. ( c ) Decrease in IL-17A and IL-17F secreting Th17 cells from CRTC2-mutant or wild-type littermates under Th17 differentiation conditions. IL-17A and IL-17F levels determined using flow cytometry. The electronic gate indicates the frequency of IL-17A (top) or IL-17F (bottom) CD4 T-cells. Data are representative of three experiments. Bar graphs represent the mean percentage (right)±s.e.m., n =3, from three independent experiments with similar results. ( d ) mRNA amounts for IL-17A, IL-17F and NR4A2 in CRTC2-mutant T-cells under Th17 differentiation conditions. Treatment with PGE 2 indicated. Data represent the mean±s.e.m.2, n =3, from three independent experiments with similar results. ( e ) Immunoblot showing effect of PGE 2 and forskolin (FSK) on CRTC2 dephosphorylation and CREB phosphorylation in CD4 T-cells under Th17 differentiation conditions. Statistical analysis were performed with unpaired Student’s t -test. Differences were considered statistically significant at P <0.05 (* P <0.05; ** P <0.005 and *** P <0.0005). Full size image Despite these effects, mRNA amounts for other Th17 genes, including the retinoic acid receptor-related orphan receptor (ROR)-yt ( rorc ), ROR-α ( rora ) and signal transducer and activator of transcription 3 ( stat3 ), were relatively unaffected by deletion of the Crtc2 gene ( Supplementary Fig. 2 ). We reasoned that loss of Crtc2 could interfere with either the proliferation or survival of Th17 cells. Supporting this notion, disruption of CREB activity has been shown to stimulate apoptosis and to reduce proliferation [16] , [17] . When placed under Th17 differentiation conditions, however, Crtc2−/− CD4 T cells showed comparable Annexin-V staining relative to wild-type cells ( Supplementary Fig. 3 ). Moreover, mRNA amounts for the anti-apoptotic factors Bcl2 and Bcl-xL appeared comparable between wild-type and Crtc2−/− cells. Arguing as well against an effect on proliferation, CRTC2-mutant CD4 T cells actually showed a slight increase in the mitotic index compared with wild type ( Supplementary Fig. 3b ). The prostaglandin PGE 2 , a product of activated innate immune cells, has been found to promote the differentiation of human and murine Th17 cells [9] . Consistent with these findings, exposure to PGE 2 stimulated CRTC2 dephosphorylation ( Fig. 1e ), and it increased il17a and il17f mRNA amounts in wild-type but not CRTC2-mutant Th17-differentiated cells ( Fig. 1d ). Exposure to PGE 2 also increased mRNA amounts for rorc , rora and stat3 , although loss of CRTC2 did not interfere with the induction of these genes ( Supplementary Fig. 4a ). Arguing against an effect on PGE 2 signalling per se , mRNA amounts for the PGE 2 receptors EP2 and EP4 were comparable between wild-type and CRTC2-mutant Th17-differentiated cells ( Supplementary Fig. 4b ). Having seen that targeted disruption of the Crtc2 gene blocks Th17 cell differentiation even in the absence of exogenous PGE 2 , we considered that T cells may themselves produce PGE 2 endogenously. Supporting this notion, T cells have been shown to express prostaglandin synthase 2 (Ptgs2) [22] . mRNA amounts for Ptgs2 were upregulated in CD4 T cells under Th17 differentiation conditions compared with undifferentiated CD4 T cells (Th0; Supplementary Fig. 4c ). Correspondingly, immunoreactive PGE 2 amounts were also increased in the medium from CD4 T cells exposed to Th17 differentiation cocktail ( Supplementary Fig. 4d ). We exposed naive CD4 T cells to individual components of the Th17 differentiation cocktail ( Supplementary Fig. 4e ). In line with its ability to stimulate Ptgs2 expression, T-cell activation by αCD3/CD28 alone was sufficient to trigger CRTC2 dephosphorylation. Although Th17 cytokines had no effect individually, exposure to a cocktail of these further enhanced effects of αCD3/CD28 on CRTC2 dephosphorylation. Together, these results indicate that endogenous PGE 2 promotes T-cell differentiation in part through the activation of CRTC2. The CREB/CRTC2 pathway regulates IL-17 expression CREB stimulates cellular gene expression by binding to palindromic (TGACGTCA) or to half site (TGACG/CGTCA) cAMP-Responsive Elements (CREs) often positioned within 1 kb of the transcriptional start site. The IL-17A gene contains two half site CREs at −144 and −54, while the IL-17F gene has half sites at −149 and at −85 relative to the transcriptional start site ( Fig. 2a ). To evaluate the potential role of CREB in mediating effects of CRTC2 on these genes, we expressed a dominant-negative CREB polypeptide called A-CREB in wild-type naive CD4 T cells under Th17 differentiation conditions. Similar to the effects we observed with loss of CRTC2, A-CREB expression significantly decreased Th17 differentiation, although to a lesser extent than CRTC2 gene disruption ( Fig. 2b , Supplementary Fig. 5 ). Consistent with their overlapping effects on CREB target genes, combined expression of A-CREB and knockout of the CRTC2 gene decreased Th17 cell differentiation more than either alone. 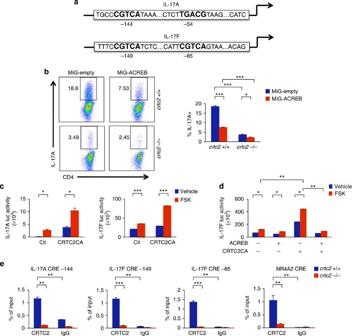Figure 2: CREB and CRTC2 regulate the expression of IL-17A and IL-17F. (a) Location of CRE sites on the mouse IL-17A and IL-17F promoters. (b) Effect of retrovirally encoded dominant-negative CREB polypeptide (ACREB) on Th17 differentiation. IL-17A levels were determined using flow cytometry. The number in each quadrant indicates the frequency of cells. Data are representative of three experiments. Bar graphs represent the mean of percentage (right)±s.e.m.,n=3, from three independent experiments. (c) Effect of phosphorylation-defective constitutively active CRTC2 on expression of IL-17A and IL-17F reporters in 293 T-cells. Effect of FSK shown. Bar graphs represent the mean of relative luciferase activity relative to co-transfectedRSVβ-gal reporter±s.e.m.,n=3, from three independent experiments. (d) Co-expression of A-CREB and constitutively active CRTC2 (CRTC2AA) on expression of IL-17A and IL-17F reporters in 293 T-cells. Bar graphs represent the mean of relative luciferase activity relative to co-transfectedRSVβ-gal reporter±s.e.m.,n=3, from three independent experiments. (e) Chromatin immunoprecipitation (ChIP) assay of sorted naive CD4 T-cells cultured under Th17 polarization conditions. Effect of PGE2on recruitment of CRTC2 to IL-17A and IL-17F promoters shown. Bar graphs represent the mean±s.e.m.,n=3, from three independent experiments. Statistical analyses were performed with unpaired Student’st-test. Differences were considered statistically significant atP<0.05 (*P<0.05; **P<0.005 and ***P<0.0005). Figure 2: CREB and CRTC2 regulate the expression of IL-17A and IL-17F. ( a ) Location of CRE sites on the mouse IL-17A and IL-17F promoters. ( b ) Effect of retrovirally encoded dominant-negative CREB polypeptide (ACREB) on Th17 differentiation. IL-17A levels were determined using flow cytometry. The number in each quadrant indicates the frequency of cells. Data are representative of three experiments. Bar graphs represent the mean of percentage (right)±s.e.m., n =3, from three independent experiments. ( c ) Effect of phosphorylation-defective constitutively active CRTC2 on expression of IL-17A and IL-17F reporters in 293 T-cells. Effect of FSK shown. Bar graphs represent the mean of relative luciferase activity relative to co-transfected RSV β-gal reporter±s.e.m., n =3, from three independent experiments. ( d ) Co-expression of A-CREB and constitutively active CRTC2 (CRTC2AA) on expression of IL-17A and IL-17F reporters in 293 T-cells. Bar graphs represent the mean of relative luciferase activity relative to co-transfected RSV β-gal reporter±s.e.m., n =3, from three independent experiments. ( e ) Chromatin immunoprecipitation (ChIP) assay of sorted naive CD4 T-cells cultured under Th17 polarization conditions. Effect of PGE 2 on recruitment of CRTC2 to IL-17A and IL-17F promoters shown. Bar graphs represent the mean±s.e.m., n =3, from three independent experiments. Statistical analyses were performed with unpaired Student’s t -test. Differences were considered statistically significant at P <0.05 (* P <0.05; ** P <0.005 and *** P <0.0005). Full size image We evaluated effects of CRTC2 on IL-17A and IL-17F promoter activity. Overexpression of phosphorylation-defective, constitutively active CRTC2 (CRTC2AA) enhanced both IL-17A and IL-17F reporters in transient transfection assays ( Fig. 2c ). Indeed, exposure to cAMP agonist forskolin further increased IL-17A and IL-17F promoter activities. In keeping with the role of CRTC2 as a CREB co-activator, co-expression of A-CREB blocked the stimulatory effects of CRTC2 in this setting ( Fig. 2d ). We performed chromatin immunoprecipitation studies to determine whether IL-17A and IL-17F genes are direct targets for CRTC2. Supporting this idea, exposure to PGE 2 increased amounts of CRTC2 over CREB-binding sites on both IL-17A and IL-17F promoters ( Fig. 2e ). Taken together, these results indicate that CRTC2 regulates IL-17A and IL-17F gene expression by binding to their promoters in response to PGE 2 stimulation. CRTC2-mutant mice are refractory to EAE Having seen that Th17 cell differentiation from naive CD4 T cells is decreased in CRTC2-mutant mice, we evaluated whether these animals would be correspondingly resistant to EAE. Following administration of immunogen (MOG 35–55 peptide), wild-type mice developed hind limb paralysis and limp tail characteristic of EAE, but CRTC2-mutant mice did not ( Fig. 3a ). Consistent with these clinical scores, Th17 cell numbers in the CNS were substantially lower in CRTC2-mutant mice compared with wild-type littermates ( Fig. 3b ). Correspondingly, spinal cord sections from CRTC2 mutants had substantially lower numbers of infiltrating cells, which were otherwise associated with demyelination ( Fig. 3c ). 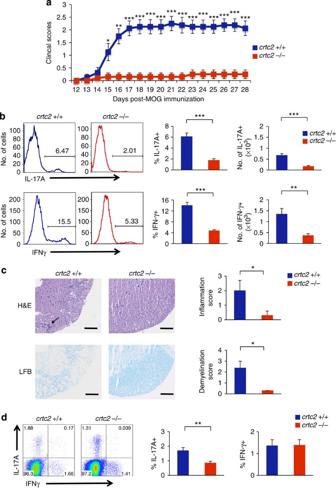Figure 3: CRTC2-mutant mice are resistant to EAE. (a) Clinical scores of wild-type and CRTC2-mutant littermates following MOG35–55immunization. Wild-type (n=8) and CRTC2-mutant (n=10) animals received 400 μg of MOG35–55peptide plus Complete Freund’s Adjuvant (CFA) on days 0 and 7 and 250 ng pertussis toxin on days 0 and 2. Each line represents the average score of the mice. Similar results were obtained in three independent studies. Data represent the mean±s.e.m. (b) Decreased Th17 cells in CRTC2-mutant mice following MOG35–55immunization. T-cells were isolated from pooled brain and spinal cord samples from mice inaon day 28 as described in Methods. T-cells were then stimulated with PMA and Ionomycin for 5 h. IL-17A (top) and IFN-γ (bottom) levels were determined using flow cytometry. Histograms are gated on live CD4 T-cells. The electronic gate indicates the frequency of IL-17A+ (top) or IFN-γ (bottom) CD4 T-cells. Bar graphs represent the mean of percentage (left) and cell numbers (right)±s.e.m.; wild-type (n=8) and CRTC2-mutant (n=10) animals. (c) The spinal cord was dissected on day 28 and stained with H&E (top) or Luxol fast blue (LFB) (bottom), and both cell infiltration and demyelination were scored. Arrow indicates infiltrating cells; scale bars, 100 μm. Bar graphs represent the mean±s.e.m.; wild-type (n=4) and CRTC2-mutant (n=5) animals. (d) Decreased Th17 cells in draining lymph nodes of CRTC2-mutant mice 7 days after MOG35–55immunization. T-cells were stimulated with PMA and Ionomycin for 5 h. Cytokine levels determined using flow cytometry. Plots are gated on live CD4 T-cells. Number in each quadrant indicates cell frequency. Bar graphs represent the mean of percentage±s.e.m.; wild-type (n=5) and CRTC2-mutant (n=5) animals. Similar results were obtained in two independent studies. Statistical analyses were performed with unpaired Student’st-test. Differences were considered statistically significant atP<0.05 (*P<0.05; **P<0.005 and ***P<0.0005). Figure 3: CRTC2-mutant mice are resistant to EAE. ( a ) Clinical scores of wild-type and CRTC2-mutant littermates following MOG 35–55 immunization. Wild-type ( n =8) and CRTC2-mutant ( n =10) animals received 400 μg of MOG 35–55 peptide plus Complete Freund’s Adjuvant (CFA) on days 0 and 7 and 250 ng pertussis toxin on days 0 and 2. Each line represents the average score of the mice. Similar results were obtained in three independent studies. Data represent the mean±s.e.m. ( b ) Decreased Th17 cells in CRTC2-mutant mice following MOG 35–55 immunization. T-cells were isolated from pooled brain and spinal cord samples from mice in a on day 28 as described in Methods. T-cells were then stimulated with PMA and Ionomycin for 5 h. IL-17A (top) and IFN-γ (bottom) levels were determined using flow cytometry. Histograms are gated on live CD4 T-cells. The electronic gate indicates the frequency of IL-17A+ (top) or IFN-γ (bottom) CD4 T-cells. Bar graphs represent the mean of percentage (left) and cell numbers (right)±s.e.m. ; wild-type ( n =8) and CRTC2-mutant ( n =10) animals. ( c ) The spinal cord was dissected on day 28 and stained with H&E (top) or Luxol fast blue (LFB) (bottom), and both cell infiltration and demyelination were scored. Arrow indicates infiltrating cells; scale bars, 100 μm. Bar graphs represent the mean±s.e.m. ; wild-type ( n =4) and CRTC2-mutant ( n =5) animals. ( d ) Decreased Th17 cells in draining lymph nodes of CRTC2-mutant mice 7 days after MOG 35–55 immunization. T-cells were stimulated with PMA and Ionomycin for 5 h. Cytokine levels determined using flow cytometry. Plots are gated on live CD4 T-cells. Number in each quadrant indicates cell frequency. Bar graphs represent the mean of percentage±s.e.m. ; wild-type ( n =5) and CRTC2-mutant ( n =5) animals. Similar results were obtained in two independent studies. Statistical analyses were performed with unpaired Student’s t -test. Differences were considered statistically significant at P <0.05 (* P <0.05; ** P <0.005 and *** P <0.0005). Full size image In principle, the decreased number of Th17 cells in the CNS of Crtc2−/− mice could reflect either a decrease in Th17 differentiation in peripheral tissues or reduced recruitment of Th17 cells into the CNS. Supporting the former, Crtc2−/− mice had fewer Th17 cells in draining lymph nodes following MOG 35–55 immunization than control littermates ( Fig. 3d ). By contrast, Th1 cell numbers were comparable between the two groups, indicating that CRTC2-mutant CD4 T cells are specifically defective in Th17 cell differentiation during induction phase of EAE. To evaluate Th17 cell recruitment to the CNS, we performed adoptive transfer experiments using MOG 35–55 -primed Th17 cells from wild-type or CRTC2-mutant mice ( Supplementary Fig. 6a ). Mice receiving Crtc2−/− Th17 cells remained refractory to EAE compared with recipient mice injected with wild-type Th17 cells ( Supplementary Fig. 6b ). Crtc2−/− Th17 cell numbers in the CNS were also decreased relative to controls ( Supplementary Fig. 6c ). By contrast, numbers of Crtc2−/− Th1 cells in the CNS were actually upregulated compared with wild type. Taken together, these data support the idea that differentiation and recruitment of Th17 cells to the CNS are both adversely affected in Crtc2−/− mice. Decreased Th17 differentiation and EAE in Crtc2 ΔCD4 mice To determine whether the effects of CRTC2 on EAE are cell-autonomous, we used the Cre–loxP system to generate mice with a deletion of CRTC2 targeted to T cells. After crossing CRTC2 fl/fl and CD4-Cre mice, we obtained Crtc2 ΔCD4 animals lacking Crtc2 expression in Th17 cells using western blot analysis ( Fig. 4a ). Similar to whole-body knockouts, Crtc2 ΔCD4 mice had normal proportions of CD4 and CD8 single-positive, double-positive and double-negative cells compared with Crtc2 fl/fl controls ( Supplementary Fig. 7a ). No differences in the proportion of T cells in the spleens of Crtc2 ΔCD4 mice were evident compared with Crtc2 fl/fl mice ( Supplementary Fig. 7b ). Percentages of effector memory (CD44hiCD62Llo) and naive (CD44loCD62Lhi) CD4+ and CD8+ T cells were also comparable between Crtc2 ΔCD4 and Crtc2 fl/fl mice ( Supplementary Fig. 7c ). 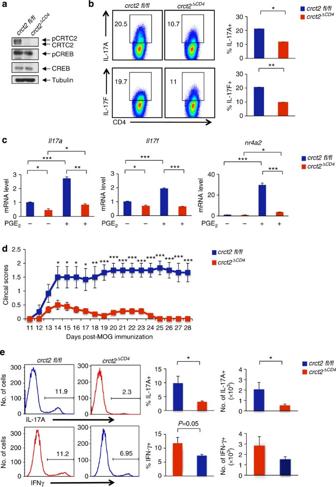Figure 4: Decreased Th17 differentiation and EAE inCrtc2ΔCD4mice. (a) Immunoblot showing CRTC2 protein amounts in control and Crtc2ΔCD4Th17 cells. (b,c) Relative differentiation of Th17 cells from CRTC2 floxedCD4creor control (CRTC2fl/fl) CD4+ T-cells. Frequency of IL-17A (top) and IL-17F (bottom) secreting Th17 cells from CRTC2-deficient or CRTC2fl/fl T-cells under Th17 differentiation conditions. Data are representative of three experiments with similar results. Bar graphs represent the mean of percentage (left) and cell numbers (right)±s.e.m.,n=3, from three independent experiments. (d)il17aandil17fmRNA amounts from CRTC2floxedCD4creT-cells under Th17 differentiation conditions. Cells treated with vehicle or PGE2 indicated. Data represent the mean±s.e.m.,n=3, from three independent experiments with similar results. (d) Crtc2ΔCD4mice are resistant to EAE. CRTC2fl/fl (n=6) and Crtc2ΔCD4(n=9) mice received 400 μg of MOG35–55peptide plus CFA on days 0 and 7, and 200 ng pertussis toxin on days 0 and 2. Mice were scored as previously described inFig. 3a. Each line represents the average score of the mice. Similar results were obtained in two independent studies. Data represent the mean±s.e.m., from two independent experiments with similar results. (e) Th17 cell numbers in the CNS of CRTC2fl/fl or Crtc2ΔCD4mice following MOG35–55immunization. Histograms are gated on live CD4+ T-cells. The electronic gate indicates the frequency of IL-17A+ (top) or IFN-γ (bottom) levels. Bar graphs represent the mean of percentage (left) and cell number (right)±s.e.m.; CRTC2 fl/fl (n=6) and Crtc2ΔCD4(n=9). Statistical analyses were performed with unpaired Student’st-test. Differences were considered statistically significant atP<0.05 (*P<0.05; **P<0.005 and ***P<0.0005). Figure 4: Decreased Th17 differentiation and EAE in Crtc2 ΔCD4 mice. ( a ) Immunoblot showing CRTC2 protein amounts in control and Crtc2 ΔCD4 Th17 cells. ( b , c ) Relative differentiation of Th17 cells from CRTC2 floxed CD4cre or control (CRTC2fl/fl) CD4+ T-cells. Frequency of IL-17A (top) and IL-17F (bottom) secreting Th17 cells from CRTC2-deficient or CRTC2fl/fl T-cells under Th17 differentiation conditions. Data are representative of three experiments with similar results. Bar graphs represent the mean of percentage (left) and cell numbers (right)±s.e.m., n =3, from three independent experiments. ( d ) il17a and il17f mRNA amounts from CRTC2floxed CD4cre T-cells under Th17 differentiation conditions. Cells treated with vehicle or PGE2 indicated. Data represent the mean±s.e.m., n =3, from three independent experiments with similar results. ( d ) Crtc2 ΔCD4 mice are resistant to EAE. CRTC2fl/fl ( n =6) and Crtc2 ΔCD4 ( n =9) mice received 400 μg of MOG 35–55 peptide plus CFA on days 0 and 7, and 200 ng pertussis toxin on days 0 and 2. Mice were scored as previously described in Fig. 3a . Each line represents the average score of the mice. Similar results were obtained in two independent studies. Data represent the mean±s.e.m., from two independent experiments with similar results. ( e ) Th17 cell numbers in the CNS of CRTC2fl/fl or Crtc2 ΔCD4 mice following MOG 35–55 immunization. Histograms are gated on live CD4+ T-cells. The electronic gate indicates the frequency of IL-17A+ (top) or IFN-γ (bottom) levels. Bar graphs represent the mean of percentage (left) and cell number (right)±s.e.m. ; CRTC2 fl/fl ( n =6) and Crtc2 ΔCD4 ( n =9). Statistical analyses were performed with unpaired Student’s t -test. Differences were considered statistically significant at P <0.05 (* P <0.05; ** P <0.005 and *** P <0.0005). Full size image Crtc2 ΔCD4 naive CD4 T cells differentiated poorly into Th17 cells relative to control ( Fig. 4b ). Under Th17 differentiation conditions, mRNA amounts for il-17a and il17f mRNA were also decreased in Crtc2 ΔCD4 CD4 T cells ( Fig. 4c ). Exposure to PGE 2 increased il17a and il17f mRNA levels in Crtc2 fl/fl but not Crtc2 ΔCD4 CD4 T cells. These results demonstrate that PGE 2 enhances il17a and il17f gene expression through induction of the CREB/CRTC2 pathway in T cells. In keeping with results from mice with a whole-body knockout of CRTC2, Crtc2 ΔCD4 mice also had significantly reduced EAE; correspondingly, CNS-infiltrating Th17 cell numbers were reduced in Crtc2 ΔCD4 mice compared with control littermates ( Fig. 4d,e ). These results indicate that the resistance to EAE in Crtc2−/− mice is intrinsic to the loss of Crtc2 expression in CD4 T cells. Although cAMP has been thought to function as a potent negative regulator of T cells [12] , we found a positive role for the CREB pathway in stimulating Th17 cell differentiation; deletion of CRTC2 selectively decreases IL-17A and IL-17F cytokine production and blocks the differentiation of naive T cells into Th17 cells ( Supplementary Fig. 8 ). In keeping with its effects on CREB and CRTC2, exposure to PGE 2 augmented the expression of both IL-17A and IL-17F genes in wild-type Th17 cells, but not in CRTC2-mutant Th17 cells. These data suggest that PGE 2 signals through the CREB/CRTC2 pathway to upregulate IL-17A and IL-17F levels and enhance Th17 cell function. PGE 2 appears to be produced both exogenously by macrophages and endogenously by differentiating T cells to activate the CREB pathway during Th17 cell differentiation. Similar to a previous study, we found that the activation of naive T cells appears sufficient to trigger Ptgs2 expression [22] . In keeping with the importance of Th17 cells for the development of autoimmune disease, CRTC2-mutant mice had significantly reduced EAE compared with wild-type mice. The resistance to EAE in CRTC2-mutant mice appears cell-autonomous because mice with targeted deletion of CRTC2 in T cells are also EAE-resistant. Although the CREB/CRTC2 pathway has been proposed to stimulate Th1 cell differentiation [23] , we were unable to detect any decrease in Th1 cell numbers or activity in the context of CRTC2 deficiency. In vivo studies also argue against a significant role for CRTC2 in Th1 cell differentiation, at least in the context of EAE. In addition to its role in T cells, the CREB/CRTC2 pathway also promotes fasting glucose homeostasis by upregulating the gluconeogenic programme in response to increases in circulating pancreatic glucagon [18] . CRTC2 activity is increased in insulin resistance, where it contributes to elevations in circulating glucose concentrations [19] . Notably, IL-17A and IL-17F expressions appear to be upregulated by elevations in glucose [24] , suggesting that the CREB pathway may also contribute to the development of autoimmune diseases in insulin resistance. Further studies should provide insight into the mechanism by which extracellular glucose modulates the expression of these cytokines. Mice C57BL/6 (B6) and CD4-Cre transgenic mice were purchased from Jackson Laboratory. CRTC2 fl/fl mice were generated by inserting the 5′ loxP site between exons 1 and 2 and placing the 3′ loxP between exons 4 and 5 (ref. 25 ). To generate Crtc2-mutant T cells, floxed Crtc2 mice were crossed to CD4-Cre mice. The CD4 T cells in the Cre + Crtc2 ΔCD4 mice were determined to be Crtc2 ΔCD4 . The wild-type littermates (Cre- Crtc2fl/fl ) were used as control ( Crtc2fl/fl ). All mice used were on a C57BL/6 background, between 6 and 12 weeks of age and sex-matched for each experiment. Mice were housed in pathogen-free conditions. Animal studies were approved and supervised by the Institutional Animal Care and Use Committee (IACUC) at the Salk Institute. Reagents Reagents were obtained as follows: PGE 2 , phorbol myristate acetate (PMA), Ionomycin and forskolin were purchased from Sigma-Aldrich; recombinant cytokines (TGF-β, IL-6, IL-7 and IL-1β) from Peprotech; IL-23 from R&D Systems; anti-CD3 (2C11), anti-CD28 (2C11), anti-IFN-γ (XMG1.2), anti-IL-12 and anti-IL-4 (11B11) antibodies were purchased from BioXCell. All antibodies used for flow cytometry were obtained from ebioscience. Tubulin antibody was purchased from Millipore. For CREB, pCREB (pSer133) and CRTC2 detection, rabbit polyclonal antibodies were raised against their respective antigens. Retrovirus MSCV-ACREB was a gift from Paul K. Brindle (St Jude’s). CD4+ T-cell isolation and differentiation in vitro CD4 T cells were isolated by immunomagnetic selection (Dynabeads FlowComp Mouse CD4 Kit, Life Technologies) from a single-cell suspension of splenocytes. Naive CD4 T cells (CD62L hi CD44 lo CD25 − ) were isolated from CD4+ T cells by cell-sorting on a FACSAria or InFlux flow cytometer (BD Biosciences). Cells were incubated with CLICKS medium (Irvine Scientific) supplemented with 2 mM l-glutamine, 100 U ml −1 penicillin, 100 μg ml −1 streptomycin, 50 μM β-mercaptoethanol and 10% FCS. Culture plates (six-well plates) were coated with anti-hamster antibody (Ab; 1:100, Vector labs). Where indicated, naive CD4 T cells were placed in supplemented CLICKS medium for 2 days after isolation to reduce background CREB phosphorylation. IL-7 was added to maintain survival of the T cells. For all differentiation conditions, naive CD4 T cells were cultured in the medium with plate-bound anti-CD3 Ab (1 μg ml −1 ) and soluble anti-CD28 (0.5 μg ml −1 ). For Th17 differentiation, cells were treated with human TGF-β (hTGF-β) (2 ng ml −1 ), IL-6 (20 ng ml −1 ), IL-1β (20 ng ml −1 ) and IL-23 (20 ng ml −1 , R&D Systems). For Th1 differentiation, cells were treated with IL-12 (20 ng ml −1 ), IL-2 (50 U ml −1 ) and anti-IL-4 (20 μg ml −1 ). For Th2 differentiation, cells were treated with IL-4 (100 U ml −1 ), anti-IL-12 (10 μg ml −1 ), IL-2 (50 U ml −1 ) and anti- IFN-γ (10 μg ml −1 ). For induced regulatory T (iTreg) generation, cells were treated with hTGF-β (5 ng ml −1 ) and IL-2 (50 U ml −1 ). For Th0, cells were treated with IL-2, in addition to the above αCD3/CD28 conditions. T cells were differentiated for 4 days, unless indicated, and then treated with PMA (50 ng ml −1 ), Ionomycin (500 ng ml −1 ) and Golgi-plug (1:1,000) for 5 h before intracellular staining. For intracellular staining, cells were fixed and permeabilized using ebioscience intracellular fixation and permeabilization kit before addition of labelled antibodies. All labelled antibodies were used at 1:300 dilutions. Cells were analysed on a LSRII flow cytometer or FACSAria. Chromatin immunoprecipitation Chromatin immunoprecipitation with CRTC2 antisera was performed as described previously [26] . Following 4 days of Th17 differentiation, Th17 cells were expanded under Th17 conditions for an additional 2 days and treated with PGE 2 (1 μM) 30 min before fixation. Cells were treated with PGE 2 at the end of Th17 differentiation to see whether PGE 2 enhanced binding of CRTC2 to CREB on the IL-17A and IL-17F promoters. Briefly, Th17 cells were fixed in 1% formaldehyde for 10 min at room temperature and then glycine (125 mM) was added to stop the crosslinking reaction for 5 min at room temperature while cells were rocking. Cells were then resuspended in cell lysis buffer (25 mM HEPES, pH 7.8, 1.5 mM MgCl 2 , 10 mM KCl, 0.3% NP-40 and 1 mM dithiothreitol) and incubated on ice for 10 min. Following 5-min centrifugation at 5,000 r.p.m., cells were resuspended in 800 μl of nuclei lysis buffer (50 mM HEPES pH 7.9, 140 mM NaCl, 1 mM EDTA, 1% Triton X-100, 0.1% Na-Deoxycholate and 0.2% SDS) and incubated on ice for 10 min. Chromatin was sonicated eight times for 15 s at level 8. Following centrifugation, supernatants were with protein A for 6 h. Supernatants were divided equally among samples and 1% was saved for input control. Two micrograms of each antibody was incubated with supernatants overnight. Protein A was then added to mix for 2 h. Following centrifugation, pellets were washed once with nucleic lysis buffer, once with nucleic lysis buffer containing 500 mM NaCl, twice with 20 mM Tris, pH 8.0, 1 mM EDTA, 250 mM LiCl, 0.5% NP-40, 0.5% Na-deoxycholate and twice with Tris EDTA (TE). The antibody/protein/DNA complexes were eluted with 1% SDS, 1 mM EDTA, 10 mM Tris, pH 8.1. Samples were then incubated at 65 °C overnight to reverse formaldehyde crosslinking. Next samples were incubated at 65 °C with proteinase K for 2 h. Glycogen was then added to the samples and DNA was extracted using phenol chloroform. Samples were resuspended in water and analysed with quantitative real-time PCR using primers listed in Supplementary Table 1 . Real-time quantitative PCR Total RNA from cells was extracted using Tripure, and cDNA was generated using the Transcriptor First Strand cDNA Synthesis kit (Roche Applied Science). cDNA was quantified on a lightcycler 480 instrument (Roche Applied Science). Gene expression data were presented relative to the expression of housekeeping gene 18s. Reporter assays HEK293T cells were cultured in DMEM (corning cellgro) containing 10% fetal bovine serum (Gemini Bio Products), 100 μg ml −1 penicillin–streptomycin and 1 mM sodium pyruvate (corning cellgro). Forskolin (10 μM) was added as indicated. HEK293T cells were transfected with lipofectamine 2,000 (Invitrogen). Luciferase activities were normalized to β-galactosidase activity. pGL4 mouse IL-17A 0.6-kb promoter plasmid was purchased from Addgene. For pGL3 mouse IL-17F promoter plasmid, 461 base pairs upstream of the mouse IL-17F start site was cloned into pGL3 using 5′-GCTCTCGAGGTGTTTAAAACCAAGTCT-3′ and 5′-GCTAAGCTTTCTCCAATGGCTGCTTCT-3′ primers. pCDNA mouse CRTC2 constitutively active (S171A, S275A) was previously described [27] . Western blot analysis Th17 cells were treated as indicated and then lysed in complete lysis buffer (150 mM NaCl, 50 mM sodium fluoride, 10 mM β-glycerophosphate, 20 mM HEPES (pH 7.4), 1% Triton X-100 with 1 mM sodium vanadate, 1 mM phenylmethylsulphonyl fluoride, 1 mg ml −1 aprotinin and 1 mg ml −1 leupeptin) and lysates were resolved on a 7.5% SDS–PAGE gel. The proteins were transferred to a polyvinylidene difluoride membrane (Immobilon-P; Millipore), prewashed in TBST and then blocked in TBST supplemented with 5% milk and incubated with primary antibody. Following an overnight incubation with the primary Ab, the blot was washed three times in TBST and incubated with peroxidase-labelled anti-rabbit secondary antibody for 1 h incubation at room temperature. To visualize western blot, the blot was washed three times in TBST, then incubated in enhanced chemiluminescence (ECL) reagent (Amersham Biosciences) and exposed to X-ray film. Images have been cropped for presentation. Full-size images are presented in Supplementary Fig. 9 . Enzyme-linked immunosorbent assays PGE 2 was quantified from Th0 or Th17 cultured cell medium. The medium without cells was used as a control. After 4 days of treatment, cells were spun down and the supernatant was collected. PGE 2 was quantified using the PGE 2 parameter assay kit from R&D Systems. Retroviral infection MSCV-IRES-GFP and MSCV-ACREB-IRES-GFP were transfected into 293T cells along with Psi-Eco packaging vector and retroviral supernatants were collected as previously described [28] . Naive CD4 T cells were differentiated into Th17 cells as stated above and infected on days 1 and 2. Fresh cytokines were added after each infection. On day 4, cells were then treated with PMA (50 ng ml −1 ), Ionomycin (500 ng ml −1 ) and Golgi-plug (1:1,000) for 5 h before intracellular staining. For intracellular staining, cells were fixed and permeabilized using ebioscience intracellular fixation and permeabilization kit before addition of labelled antibodies. Active EAE On days 0 and 7 mice were immunized with 400 μg of MOG 35–55 peptide supplemented with complete Freund’s adjuvant containing 4 mg ml −1 dessicated tuberculosis. On days 0 and 2 mice were injected with 250 ng of pertussis toxin (List Biologicals). Mice were monitored daily for signs of clinical disease following EAE induction using the following scale: (0.5) altered gait and/or hunched appearance, (1) limp tail, (2) partial hind limb paralysis, (3) complete hind limb paralysis, (4) complete hind limb paralysis and partial fore limb paralysis and (5) death. Passive EAE On day 0, donor mice were immunized with 400 μg of MOG 35–55 supplemented with complete Freund’s adjuvant containing 4 mg ml −1 desiccated tuberculosis. On day 10, draining lymph nodes were harvested and cells were cultured at 5 million cells ml −1 under Th17 differentiation conditions in addition to 20 μg ml −1 of MOG 35–55 peptide. On day 14, cells were restimulated at 2 million cells ml −1 using plate-bound anti-CD3 and soluble anti-CD28 antibodies in the presence of 20 ng ml −1 IL-18. On day 15, 4–5 million cells were injected intraperitoneally into sublethally irradiated mice. To compensate for the decrease in Th17 differentiation, recipients receiving CRTC2-mutant cells received 5 million cells instead of the 4 million cells that the wild-type recipients received. Mice were monitored daily for signs of clinical disease following EAE induction using the same scale as in active EAE. Leukocyte isolation from the CNS At the end of EAE, mice were killed and their brains and spinal cords were collected. Brains and spinal cords were pooled and treated with 2 mg ml −1 of collagenase and 10 units of Dnase for 30 min at 37 °C. Samples were then filtered through a 70-μm nylon mesh and leukocytes were isolated through a Percoll gradient. Leuokocytes were then treated with PMA (50 ng ml −1 ), Ionomycin (500 ng ml −1 ) and Golgi-plug (1:1,000) for 5 h before intracellular staining. For intracellular staining, cells were fixed and permeabilized using ebioscience intracellular fixation and the permeabilization kit before addition of labelled antibodies. Evaluation of the spinal cord sections Spinal cords were dissected on day 28 and stained with haematoxylin and eosin (H&E) or Luxol fast blue, and both cell infiltration and demyelination were scored. H&E slides were assessed for inflammation using the following scoring system: (0)=no evidence of inflammation; (1) rare, scattered small foci of cellular inflammation; (2) multiple, isolated foci of cellular infiltration; (3) multiple, confluent foci of inflammation; and (4) foci of necrosis and/or neutrophilic infiltration. Luxol fast blue slides were assessed for neuronal degeneration or axonal swelling using the following scoring system: (0) normal; (1) minimal or few, scattered degenerative neurons; (3) moderate, multifocal groups of degenerative neurons; (3) marked or large, multifocal degenerative neurons; and (4) severe or coalescing groups of degenerative neurons. Statistical analysis All mice used in experiments were ∼ 6–12 weeks old. Whenever possible, littermates of appropriate genotypes were used as age- and sex-matched controls. The number of mice per experiment was limited by the availability of the required genotype and age. Criteria of exclusion were: (1) age, (2) evident signs of disease and (3) spontaneous natural death during the experiment. Sample size (number of mice, spleens and cells) is within the range of published unless indicated. Statistical analyses were performed with unpaired Student’s t -test. Differences were considered statistically significant at P <0.05 (* P <0.05; ** P <0.01 and *** P <0.001). How to cite this article: Hernandez, J.B. et al . The CREB/CRTC2 pathway modulates autoimmune disease by promoting Th17 differentiation. Nat. Commun. 6:7216 doi: 10.1038/ncomms8216 (2015).